Template-mediated nano-crystallite networks in semiconducting polymers Unlike typical inorganic semiconductors with a crystal structure, the charge dynamics of π-conjugated polymers (π-CPs) are severely limited by the presence of amorphous portions between the ordered crystalline regions. Thus, the formation of interconnected pathways along crystallites of π-CPs is desired to ensure highly efficient charge transport in printable electronics. Here we report the formation of nano-crystallite networks in π-CP films by employing novel template-mediated crystallization (TMC) via polaron formation and electrostatic interaction. The lateral and vertical charge transport of TMC-treated films increased by two orders of magnitude compared with pristine π-CPs. In particular, because of the unprecedented room temperature and solution-processing advantages of our TMC method, we achieve a field-effect mobility of 0.25 cm 2 V −1 s −1 using a plastic substrate, which corresponds to the highest value reported thus far. Because our findings can be applied to various π-conjugated semiconductors, our approach is universal and is expected to yield high-performance printable electronics. Printable electronics, which utilize π-conjugated semiconducting and metallic polymers (π-CPs) as electronic inks, are emerging as a promising technology for the low-cost production of flexible and lightweight devices for use in future ubiquitous devices [1] , [2] , [3] , [4] . However, the device performance of π-CPs remains inferior to that of their inorganic counterparts. In contrast to the well-aligned and highly crystalline structure of conventional semiconductors, in which three-dimensional (3D) band-diffusion transport enables high charge-carrier mobility, the charge dynamics in π-CPs are mostly limited by the structure disorder and/or the amorphous portions at the mesoscopic length scale [5] , [6] , [7] , [8] . Therefore, the formation of interconnected pathways along the crystallites of π-CPs is desired to ensure highly efficient long-range charge transport in printable electronics. Because the ultimate advantage of π-CPs is to fabricate devices from solution on top of plastic substrates, inducing interconnected crystallite structures from π-CP solutions at room temperature (RT) is a challenge. Because π-CP chains exhibit a high degree of conformational disorder and weakly interact with each other through van der Waals forces (<10 kcal mol −1 ) in their solution state, amorphous regions and ordered regions are highly likely to statistically coexist in cast π-CP films. The characteristic chain-entangled structure of the amorphous regions hinders the delocalization of the π-electron wave functions in π-CPs. To reduce the amorphous regions and thereby extend the ordered structure of π-CPs, substantial progress has recently been made in the molecular design and fabrication of π-CP films with an impressive field-effect mobility ( μ FET ) that exceeds 6 cm 2 V −1 s −1 (refs 9 , 10 , 11 , 12 , 13 ). However, the high-T processing (typically, T ⩾ 200 °C) and the rigid substrates of these techniques are critical factors that limit their application to flexible and printable technologies that utilize plastic substrates. Recent important developments in polymer field-effect transistors (PFETs) with rigid substrates based on mechanical rubbing [14] , [15] and/or solvent-induced directional solidification [16] using grooved substrates [11] , [17] , [18] are not applicable to newer plastic electronics that use flexible and printable techniques. In addition, because these alignment techniques induce enhanced charge transport ( μ FET ⩾ 6 cm 2 V −1 s −1 ) only in the lateral direction, these one-dimensional anisotropic systems [11] , [12] , [13] , [14] , [15] , [16] , [17] , [18] limit their general use in plastic electronics, which require not only lateral charge transport as in PFETs but also vertical charge transport as in polymer solar cells [19] and polymer light-emitting diodes [20] . Therefore, prior to this report, no true interconnected pathway of π-CP with 3D network formation from solution at RT had been demonstrated. In this work, we report the observation of the structural formation of crystallite-fibril nanostructures and interconnected networks in solution-processed π-CP films fabricated using a template-mediated crystallization (TMC) method at RT. By employing a polymer template incorporated with periodically repeating sulphonic acid side-chain groups, such as poly(4-styrene sulphonic acid) (PSS) [21] , π-CPs were crystallized along the PSS template to form a microscale fibril structure via polaron formation and electrostatic interaction between π-CPs and the side chain of PSS. Consequently, the template-mediated fibril structures with light doping are physically interconnected with long-range order, leading to 3D percolation networks in the π-CP films. Therefore, the μ FET values of our TMC-treated π-CP films dramatically increased by one or two orders of magnitude compared with those of the pristine π-CPs without any extra treatments. Additionally, because of the well-connected electrical percolation system within the film, our systems exhibit 3D isotropic transport with the same order of improvement along the vertical and lateral directions. Solution preparation and TMC reaction The chemical structure of a π-CP (here poly(3-hexylthiophene-2,5-diyl), (P3HT)) [22] , [23] and PSS are shown in Fig. 1a . After preparing two pristine P3HT solutions (10 mg ml −1 ) by dissolution in a chloroform solvent, we added 10 mg of PSS into one of the P3HT solutions and stirred for more than 3 days (see Methods and Supplementary Fig. 1a and Supplementary Note 1 for more details). All of the sample preparation conditions were identical except for the addition of PSS into one of the samples. We subsequently observed that the TMC reaction of P3HT was initiated along the PSS template. Initial evidence of the P3HT crystallization via TMC was observed in the ultraviolet–visible absorption spectra ( Fig. 1a ), which exhibited a considerable increase in the 0–0 vibronic transition at 600 nm [24] and in the polaron transition at 1,000 nm [25] , [26] for the PSS-added solution and film samples (that is, P3HT:PSS). We also observed a distinct electron spin resonance (ESR) signal for the P3HT:PSS (1:1 w/w) solution in the dark at RT, whereas no ESR signal was observed in the pristine P3HT and pure PSS solutions ( Fig. 1b ). The 1,000 nm absorption feature and the ESR signal of P3HT:PSS provide strong evidence of the presence of radical cations (spin 1/2) on P3HT (P3HT +· ), which are associated with a lattice distortion known as a polaron state [26] (see the chemical structure in the inset of Fig. 1b ). We consider the P3HT + cations to be stabilized by the anions of the PSS template via an electrostatic interaction [21] , [27] , resulting in a new fibril microstructure, as evident in the phase-mode atomic force microscopy (AFM) image of the P3HT:PSS films ( Supplementary Fig. 1b ). To probe the doping mechanism and the presence of electrostatic interaction between P3HT and PSS, X-ray photoelectron spectroscopy (XPS) measurement was performed on the P3HT and P3HT:PSS films, as shown Fig. 1c . The XPS spectra acquired in the sulphur region of the P3HT and P3HT:PSS films were deconvoluted into two doublets. The doublet peaks in the P3HT film (black line, solid) located at 163.9 and 165.1 eV could be assigned to the sulphur of thiophene [27] , whereas the doublet peaks in the P3HT:PSS film (blue line, solid) were located at 164.1 and 165.3 eV, indicating that the sulphur of thiophene would be positively charged [27] , [28] . In addition, comparing the doublet peaks in the pristine PSS film (unionized sulphonic acid group) located at 169.0 and 170.3 eV ( Supplementary Fig. 2 ) revealed that the doublet peaks of the P3HT:PSS film were slightly shifted towards low binding energy at 168.1 and 169.5 eV, as shown in the inset, which are assigned to the ionized sulphonic acid groups (−SO3 − ) of PSS [27] . From the XPS results, we suggest that the P3HT could be protonated to carry a positive charge on sulphur, which would be electrostatically associated with the ionized SO 3 − of PSS. 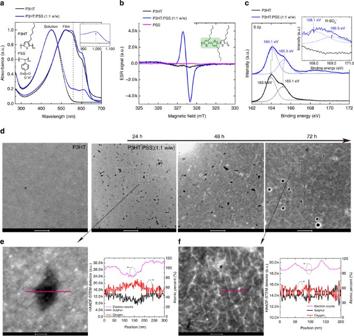Figure 1: Characterization of the template-mediated crystallization of P3HT. (a) Ultraviolet–visible absorption spectra of the P3HT and P3HT:PSS solutions (dots) and films (solids). The inset presents the absorption spectra at 1,000 nm (1.3 eV), where a polaron transition occurs. (b) ESR spectra of the pristine P3HT, PSS and P3HT:PSS solutions. The g-factor is 1.9999. (c) X-ray photoemission spectroscopy (XPS) of the corresponding films. The slightly shifted binding energy of sulphur in the P3HT:PSS film (blue line) indicates the presence of positively charged sulphur. The inset reveals the presence of ionized PSS−in the P3HT:PSS film. (d) The sequential change of the nanomorphology of the P3HT:PSS film as a function of time (from 0 to 72 h) using high-angle annular dark-field scanning TEM (HAADF-STEM). Scale bars, 1 μm. (e,f) Electron dispersive spectroscopy on the selected region of the P3HT:PSS film after 24 h and the P3HT:PSS film after 72 h, respectively. Scale bars, 100 nm. Figure 1: Characterization of the template-mediated crystallization of P3HT. ( a ) Ultraviolet–visible absorption spectra of the P3HT and P3HT:PSS solutions (dots) and films (solids). The inset presents the absorption spectra at 1,000 nm (1.3 eV), where a polaron transition occurs. ( b ) ESR spectra of the pristine P3HT, PSS and P3HT:PSS solutions. The g-factor is 1.9999. ( c ) X-ray photoemission spectroscopy (XPS) of the corresponding films. The slightly shifted binding energy of sulphur in the P3HT:PSS film (blue line) indicates the presence of positively charged sulphur. The inset reveals the presence of ionized PSS − in the P3HT:PSS film. ( d ) The sequential change of the nanomorphology of the P3HT:PSS film as a function of time (from 0 to 72 h) using high-angle annular dark-field scanning TEM (HAADF-STEM). Scale bars, 1 μm. ( e , f ) Electron dispersive spectroscopy on the selected region of the P3HT:PSS film after 24 h and the P3HT:PSS film after 72 h, respectively. Scale bars, 100 nm. Full size image Formation of crystallite-fibril nanostructure in the P3HT:PSS film We observed that the P3HT and PSS continued to develop the TMC formation for more than 72 h ( Supplementary Fig. 1 ). To monitor the progress of formation of the TMC nanostructure, we sequentially characterized the nanomorphology of the P3HT:PSS film as a function of time using high-angle annular dark-field scanning transmission electron microscopy (HAADF-STEM) ( Fig. 1d ). The pristine P3HT did not exhibit any relevant features. Notably, however, we could identify randomly distributed, irregular-shaped dark spots ranging from 50 to 500 nm (after 24 h). An electron dispersive X-ray spectroscopy (EDS) line-profile analysis on the dark region of P3HT:PSS film (after 24 h) revealed that the composition of oxygen is relatively higher compared with that of sulphur, suggesting the presence of insulating PSS because the specific atoms of the P3HT single unit are almost identical to those of PSS except the presence of oxygen atoms in the former ( Fig. 1e ). Because the PSS chemically reacts with the P3HT during the TMC formation, we hypothesized that the PSS region might decrease as the TMC-induced fibril nanomorphology developed as a function of time. Indeed, the dark regions were gradually reduced, whereas the evolution of the fibrillar structure was observed in the entire P3HT:PSS film after 48 h. Eventually, the final TMC-induced fibril network nanomorphology on the scale of ~10–20 nm in width and 1–2 μm in length throughout the entire film was formed in the film after 72 h. The sequential change in the nanomorphology of the P3HT:PSS film indicated that the PSS served as a template for forming the TMC-induced fibrillar structure. In addition, because the electron dispersive X-ray spectroscopy line profile on the TMC-induced fibril structure did not show a clear sulphur/oxygen compositional variation ( Fig. 1f ), we anticipate that the indistinguishable amount of the PSS template may coexist with the P3HT in the fibril structure, which consists of P3HT:PSS. In contrast to diffraction contrast TEM imaging, which uses coherent elastic scattered electrons, the HAADF-STEM images is obtained from incoherently scattered electrons, which are highly sensitive to variations in the atomic number of atoms and/or relative differences in the electron density of the sample [29] . Thus, the brighter regions in the HAADF-STEM image would be attributed to a relatively higher electron density of the fibrillar structure than that of the surrounding regions. Therefore, we speculate that the TMC-induced fibrillar network nanostructure (after 72 h, Fig. 1d ) could have originated from the P3HT molecules that are highly packed and oriented. Structural evolution and 3D electrical percolation network To investigate the improved structural orientation of the P3HT:PSS films, we performed grazing-incidence wide-angle X-ray scattering (GIWAXS) measurements [30] , [31] , [32] on the P3HT and P3HT:PSS films (see Methods for further details). 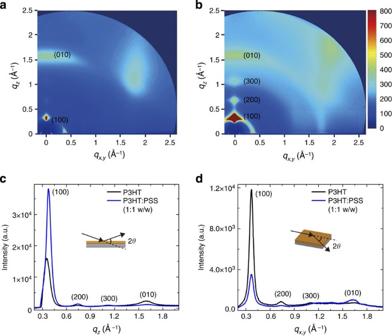Figure 2: GIWAXS investigations of P3HT and P3HT:PSS (1:1 w/w) films. (a,b) Two-dimensional GIWAXS from the pristine P3HT and P3HT:PSS (1:1 w/w) films on a silicon wafer. The incident angle was selected as 0.6°. (c,d) One-dimensional scattering profiles (out-of-plane and in-plane directions, respectively) obtained from the two-dimensional GIWAXS images. The insets show the incident direction of the X-ray beam. Figure 2a,b present two-dimensional GIWAXS profiles of the pristine P3HT and the P3HT:PSS films. For the pristine P3HT film, two diffusive elliptical-like patterns were observed along the out-of-plane direction at q z (Å −1 )=0.366, which is associated with a lamellar spacing of the (100) plane (2π/0.366=17.2 Å) and at q z (Å −1 )=1.59, which corresponds to the π–π stacking distance of the (010) plane (2π/1.59=3.95 Å). In contrast, the peak associated with the in-plane direction appears at q x , y (Å −1 )=0.37, with a weak diffusive elliptical-like pattern. Thus, the weak ‘face-on’ direction is more favourable in the pristine P3HT film, which implies that lateral charge transport is limited in the pristine P3HT films. For the P3HT:PSS films, however, a series of intense spots appear at the peak positions for the ( h 00) plane along the q z axis. In addition, an arcing shape for the π–π stacking of the (010) plane along both the q z axis and the q x , y axis was developed. More importantly, we observed two reverse trends of intensity, one at q z (Å −1 )=0.37 and 1.60 and another at q x , y (Å −1 )=0.37 and 1.60, in the one-dimensional scattering profile of the P3HT and the P3HT:PSS films, as shown in Fig. 2c,d , respectively. These results indicate an evolution of the ‘edge-on’ orientation in the P3HT:PSS films and the overall enhancement of in-plane π–π stacking for the lateral charge transport [33] , [34] . Figure 2: GIWAXS investigations of P3HT and P3HT:PSS (1:1 w/w) films. ( a , b ) Two-dimensional GIWAXS from the pristine P3HT and P3HT:PSS (1:1 w/w) films on a silicon wafer. The incident angle was selected as 0.6°. ( c , d ) One-dimensional scattering profiles (out-of-plane and in-plane directions, respectively) obtained from the two-dimensional GIWAXS images. The insets show the incident direction of the X-ray beam. Full size image The relationship between the changed structural formation and the electrical performance for the TMC-induced nanostructure film was investigated using conducting-probe AFM [35] , [36] . We measured the contact current on the pristine P3HT and P3HT:PSS films by applying a negative bias ( V bias =−5 V) to a Pt/Cr-coated tip (the Au electrode was grounded). As observed in the topographic images of the two films ( Fig. 3a,b ), the P3HT:PSS film exhibited a rougher surface morphology with a clearer fibril structure compared with the P3HT film. Surprisingly, these morphological changes are more evident in the current images. In the pristine P3HT film, grain-shaped bright regions (high current) with a diameter that varies between 200 nm and 1 μm were observed. Note that these bright regions are surrounded by dark regions (low current). Thus, it is clear that the lateral charge transport across the entire pristine P3HT film is severely limited by the grain boundary. However, in the P3HT:PSS film, these bright regions are interconnected and spread out throughout the entire film. In addition, the contact current value in the P3HT:PSS film increases by two orders of magnitude compared with that of the pristine P3HT film (see Fig. 3c , the corresponding histograms of the current images of the two films). Because conducting-probe AFM can measure local charge transport in the vertical direction, these results indicate that the vertical charge transports are also enhanced. This observation is consistent with the time-of-flight (ToF) measurements, which are a typical tool used for measuring the vertical transport of semiconductors, on the Indium tin oxide (ITO)/P3HT/Al and ITO/P3HT:PSS/Al device configuration [3] , [37] , [38] . The measurement was performed at 532 nm using the frequency-doubled outputs of a Nd:YAG laser (LOTIS). The ToF transients of the P3HT and P3HT:PSS devices were measured at 20–200 V applied biases under pulsed (5 ns) illumination through the ITO electrode. Fig. 3d,e show the typical hole current transient of the P3HT ( t ~10 μm) and P3HT:PSS films ( t ~13 μm) devices recorded at E=2.0 × 10 5 V cm −1 and 1.6 × 10 4 V cm −1 , respectively. The data are plotted on a log–log scale (main plot); the transit time, t tr , is denoted with an arrow and is estimated from the intersection point of the log–log plot. The ToF mobility of the P3HT device of ~5 × 10 −4 cm 2 V −1 s −1 at E=2 × 10 5 V cm −1 is very similar to that observed in previous studies. However, the ToF mobility in the P3HT:PSS device is remarkably improved by almost two orders of magnitude: ~1.4 × 10 −2 cm 2 V −1 s −1 at E=1.6 × 10 4 V cm −1 . We also consistently observed the mobility of the P3HT and P3HT:PSS films ( t ~130 nm) in the space-charge-limited current regime ( Supplementary Fig. 3 and Supplementary Note 2 ). Therefore, we concluded that the crystallite-fibril nanostructure and network formation in the P3HT:PSS film induce well-connected, 3D, and isotropic percolation networks for charge transport. 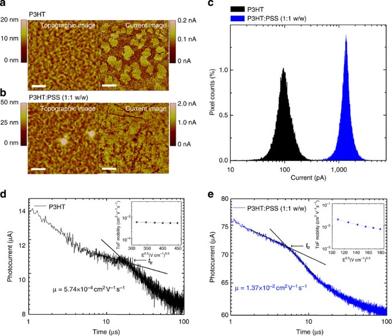Figure 3: Relationship between the film morphology and electrical performance. (a,b) Conducting-probe AFM images of P3HT and P3HT:PSS (1:1 w/w) films. Scale bars, 1 μm. (c) Current histograms of P3HT and P3HT:PSS (1:1 w/w) films obtained from the corresponding current image. (d,e) Transient photocurrent from time-of-flight (ToF) measurements with a device geometry of ITO/P3HT/Al and ITO/P3HT:PSS/Al, respectively. The insets indicate the hole mobility of the corresponding devices plotted as a function of the square root of various bias fields. Figure 3: Relationship between the film morphology and electrical performance. ( a , b ) Conducting-probe AFM images of P3HT and P3HT:PSS (1:1 w/w) films. Scale bars, 1 μm. ( c ) Current histograms of P3HT and P3HT:PSS (1:1 w/w) films obtained from the corresponding current image. ( d , e ) Transient photocurrent from time-of-flight (ToF) measurements with a device geometry of ITO/P3HT/Al and ITO/P3HT:PSS/Al, respectively. The insets indicate the hole mobility of the corresponding devices plotted as a function of the square root of various bias fields. Full size image Role of doping and template agents in π-CP films From a series of optical, structural and electrical experiments on the π-CPs:PSS films, we observed that the acid side-chain group (R-SO 3 H) of PSS enables the doping process on π-CP films, whereas the polymer backbone of PSS serves as a structural template for the molecular orientation of π-CPs with a TMC-induced fibril nanostructure. Such bifunctional behaviour of PSS must be related to high-performance electronics of the π-CPs:PSS film. To clarify the relationship between the doping process and the action as a template, we performed experiments using various types of doping/template agents as illustrated in Fig. 4a . We hypothesized that acidic molecular dopants (red panel), such as p-toluene sulphonic acid (TSS) and methanesulfonic acid (MSA), only have a single function of chemical doping on π-CPs (that is, P3HT), whereas non-acidic polymer template agents (green panel), such as poly(sodium 4-styrene sulphonate) (PSS − :Na + ) and polystyrene (PS), only serve as a template for the molecular orientation of π-CPs. Further information on P3HT:MSA and P3HT:PS films can be found in Supplementary Figs 4 and 5 and Supplementary Table 1 . 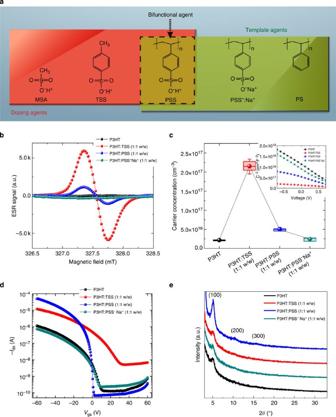Figure 4: Role of doping and template agents in π-CP films. (a) Schematic diagram of the categorization of doping and template agents depending on their chemical structure. The acidic molecules of MSA and TSS shown in the red panel and the non-acidic polymer of PSS−:Na+and PS in the green panel are the doping agents and template agents, respectively; PSS is categorized in the intersection region and is called the bifunctional agent. (b) ESR spectra of the pristine P3HT, P3HT:TSS, P3HT:PSS and P3HT:PSS−:Na+solutions. (c) Plot of charge-carrier density of the corresponding films measured in typical M-I-M configuration, ITO/semiconductor/aluminium. The inset presents a Mott–Schottky plot of the films. The error bars represent standard deviations derived from more than three devices. (d) Transfer characteristics of the corresponding PFETs on a Si++/SiO2silicon wafer (tox~200 nm); the charge-carrier mobility of the P3HT:TSS film is on the order of ~0.01 cm2V−1s−1, whereas the mobility of P3HT:PSS−:Na+is on the order of ~0.001 cm2V−1s−1. (e) High-resolution X-ray diffraction (HR-XRD) patterns of the corresponding films. Figure 4: Role of doping and template agents in π-CP films. ( a ) Schematic diagram of the categorization of doping and template agents depending on their chemical structure. The acidic molecules of MSA and TSS shown in the red panel and the non-acidic polymer of PSS − :Na + and PS in the green panel are the doping agents and template agents, respectively; PSS is categorized in the intersection region and is called the bifunctional agent. ( b ) ESR spectra of the pristine P3HT, P3HT:TSS, P3HT:PSS and P3HT:PSS − :Na + solutions. ( c ) Plot of charge-carrier density of the corresponding films measured in typical M-I-M configuration, ITO/semiconductor/aluminium. The inset presents a Mott–Schottky plot of the films. The error bars represent standard deviations derived from more than three devices. ( d ) Transfer characteristics of the corresponding PFETs on a Si ++ /SiO 2 silicon wafer ( t ox ~200 nm); the charge-carrier mobility of the P3HT:TSS film is on the order of ~0.01 cm 2 V − 1 s − 1 , whereas the mobility of P3HT:PSS − :Na + is on the order of ~0.001 cm 2 V − 1 s − 1 . ( e ) High-resolution X-ray diffraction (HR-XRD) patterns of the corresponding films. Full size image Figure 4b reveals that distinct ESR signals were observed for the P3HT:TSS and P3HT:PSS films even though no relevant features were observed in the pristine P3HT and P3HT:PSS − :Na + films , implying that the doping process would only be induced by the protonation of acidic dopants. Figure 4c demonstrates the change of charge-carrier density in the corresponding films. The inset presents Mott–Schottky plots ( C −2 versus V ) of the films. As expected, little change was observed in the charge-carrier density for the P3HT:PSS − :Na + film compared with that of the P3HT film (~2.0 × 10 16 cm −3 ). However, we observed that the P3HT:PSS film was lightly doped to have a charge-carrier density of 4.6 × 10 16 cm −3 , whereas the P3HT:TSS film was moderately doped to have a charge-carrier density of 2.2 × 10 17 cm −3 , which is an order of magnitude higher than that of the P3HT film. This behaviour might be interpreted as suggesting the possibility of a light and moderate doping effect on the corresponding transistor performances [39] , [40] , [41] . To verify the doping effect on the transistor performance, the transfer characteristics with a bottom-gate and top-contact transistor configuration ( L =50 μm, W =1,000 μm) for the corresponding films were determined as shown in Fig. 4d . Although the P3HT:TSS transistor exhibited a field-effect mobility on the order of ~10 −2 cm 2 V −1 s −1 but a reduced on/off ratio (~10 3 ) with the threshold voltage shifting towards positive values, the P3HT:PSS transistor exhibited a high field-effect mobility (~10 −1 cm 2 V −1 s −1 ) and a high on-off ratio (~10 6 ) without any threshold shift. This result implied that the light doping process on P3HT would help to extend the electrical connectivity and minimize the trap sites, leading to high-performance electronics [41] . We further noted that the P3HT:TSS film did not exhibit the TMC nanomorphology or the interconnected network that were clearly observed in the P3HT:PSS film, suggesting that the molecular dopant could not serve as a template for the structural orientation ( Supplementary Fig. 6 ). A consistent result was observed in the high-resolution X-ray diffraction spectra of the corresponding films in Fig. 4e . No structural change was observed in either the doped P3HT:TSS film or the undoped P3HT:PSS − :Na + film compared with the P3HT film, whereas a distinct X-ray peak at the (100) plane was observed in the lightly doped P3HT:PSS film. Therefore, by monitoring the change in the charge-carrier density, structural orientation and electrical properties of the P3HT film associated with the various doping/template agent, we concluded that the bifunctional agent (that is, PSS) incorporated with the acid side-chain groups and template polymer backbone would substantially contribute to the light doping process and the structural orientation, thereby leading to a high-performance device exhibiting a high on-current and low off-current. Hole mobilities in the π-CPs:PSS films at RT Using a combination of the light doping effect and structural enhancement of π-CPs induced by the bifunctional agent, PSS, we fabricated PFETs to investigate the hole transport characteristics across various π-CPs:PSS films. The PFETs ( L =50 μm and W =1,000 μm, defined by a Au source/drain electrode) were fabricated on a heavily n-doped silicon/SiO 2 ( t ox =200 nm) substrate with a bottom-gate and top-contact configuration. Note that the transistors were fabricated without any additional process such as a self-assembled monolayer [9] or high-temperature process (>150 °C) [10] , which are typically required for the manipulation of the oriented structure in π-CPs. In Fig. 5a , the pristine P3HT exhibits a relatively low average μ FET ≈8.8 × 10 −4 cm 2 V −1 s −1 with an on/off ratio of 10 4 . However, after the PSS template polymer is added to P3HT, the μ FET value dramatically increases to an average μ FET ≈0.1 cm 2 V −1 s −1 (the maximum μ FET ≈0.18 cm 2 V −1 s −1 ) with an on/off ratio of ~10 6 and an excellent shelf-life stability [41] , [42] (additional information is provided in Supplementary Figs 7 and 8 and Supplementary Notes 3 and 4 ). Using the gated transmission line model [43] , [44] , we also observed that the channel resistance of the P3HT:PSS transistor is two orders of magnitude lower than that of the pristine P3HT transistor ( Supplementary Fig. 9 and Supplementary Notes 5 ). We also applied our TMC method to other π-conjugated semiconductors containing a thiophene unit, such as poly[2,5-bis(alkyl)pyrrolo[3,4-c]pyrrole-1,4(2 H ,5 H )-dione- alt -5,5′-di(thiophen-2-yl)-2,2′-( E )-2-(2-(thiophen-2-yl)vinyl)thiophene](PDVT-10) polymers [45] and 5,5′-bis[(4-(7-hexylthiophen-2-yl)thiophen-2-yl)-[1,2,5]thiadiaz-olo[3,4-c]pyridine]-3,3′-di-2-ethylhexylsilylene-2,2′-bithiophene (DTS(PTTh 2 ) 2 ) small molecules [46] , [47] . As demonstrated in Fig. 5b , the PDVT-10:PSS (1:1 w/w) transistor exhibits an average mobility of 0.8 cm 2 V −1 s −1 (the maximum μ FET ≈1.1 cm 2 V −1 s −1 ), with a reasonable on/off ratio of ~10 6 , which is an order of magnitude higher than that of the pristine PDVT-10 transistor (~0.13 cm 2 V −1 s −1 ). Similar trends were also observed in the DTS(PTTh 2 ) 2 :PSS (1:0.2 w/w) transistor ( Fig. 5c ); the average mobility increased by an order of magnitude (from 0.03 cm 2 V −1 s −1 to 0.27 cm 2 V −1 s −1 ), with an on/off ratio of ~10 7 (see Supplementary Fig. 10 for more details). Although the optimized PSS template ratio for the highest device performance was different for each material, we concluded that our PSS template method clearly improves the charge transport of the various π-CPs semiconductors through a combination of the template-mediated structural evolution and light doping effect ( Supplementary Figs 11 and 12 ). 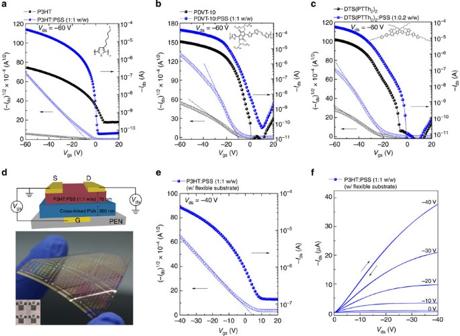Figure 5: High-performance OFET devices with various π-CPs:PSS films. (a) Transfer characteristics of OFETs on a heavily n-doped Si/SiO2silicon wafer (tox~200 nm) using P3HT semiconductors with and without the PSS template; the OFETs exhibit an improved charge-carrier mobility from 0.0009, cm2V−1s−1to ~0.18 cm2V−1s−1. (b,c) Transfer characteristics of OFETs on Si++/SiO2silicon wafers (tox~200 nm) using PDVT-10 and DTS(PTTh2)2with and without the PSS template; the OFETs exhibit an improved charge-carrier mobility from 0.1 cm2V−1s−1to 1.1 cm2V−1s−1for PDVT-10 and from 0.03 cm2V−1s−1to 0.27 cm2V−1s−1for DTS(PTTh2)2, respectively. The insets show the respective chemical structures. (d) The schematic device structure and an image of the corresponding flexible PFETs with an area of 4.4 × 4.4 cm2(324 devices). (e) Transfer characteristics of the flexible PFET devices with the P3HT:PSS film (1:1 w/w); the devices exhibit a saturation-regime mobility of ~0.25 cm2V−1s−1. (f) Output characteristics of the flexible PFET devices with the P3HT:PSS film (1:1 w/w). Figure 5: High-performance OFET devices with various π-CPs:PSS films. ( a ) Transfer characteristics of OFETs on a heavily n-doped Si/SiO 2 silicon wafer ( t ox ~200 nm) using P3HT semiconductors with and without the PSS template; the OFETs exhibit an improved charge-carrier mobility from 0.0009, cm 2 V − 1 s − 1 to ~0.18 cm 2 V − 1 s − 1 . ( b , c ) Transfer characteristics of OFETs on Si ++ /SiO 2 silicon wafers ( t ox ~200 nm) using PDVT-10 and DTS(PTTh 2 ) 2 with and without the PSS template; the OFETs exhibit an improved charge-carrier mobility from 0.1 cm 2 V − 1 s − 1 to 1.1 cm 2 V − 1 s − 1 for PDVT-10 and from 0.03 cm 2 V − 1 s − 1 to 0.27 cm 2 V − 1 s − 1 for DTS(PTTh 2 ) 2 , respectively. The insets show the respective chemical structures. ( d ) The schematic device structure and an image of the corresponding flexible PFETs with an area of 4.4 × 4.4 cm 2 (324 devices). ( e ) Transfer characteristics of the flexible PFET devices with the P3HT:PSS film (1:1 w/w); the devices exhibit a saturation-regime mobility of ~0.25 cm 2 V − 1 s − 1 . ( f ) Output characteristics of the flexible PFET devices with the P3HT:PSS film (1:1 w/w). Full size image To demonstrate the merits of our TMC method, we successfully produced large-area flexible PFETs fabricated on top of plastic substrates with P3HT:PSS. Figure 5d shows the device configuration and presents an image of the large-area flexible PFET (4.4 × 4.4 cm 2 ). As observed in Fig. 5e,f , the flexible PFETs exhibited an average μ FET of ~0.14 cm 2 V −1 s −1 (the maximum μ FET ≈0.25 cm 2 V −1 s −1 ), which is two orders of magnitude greater than that of the pristine P3HT (~0.001 cm 2 V −1 s −1 ) and corresponds to the highest μ FET value reported thus far in the devices fabricated on the plastic substrates without any additional steps. Proposed mechanism for TMC formation in π-CPs:PSS film Based on our results, the mechanism of light doping and TMC formation in the π-CPs:PSS film (that is, P3HT:PSS) is suggested in Fig. 6a . PSS is a linear polymer with periodically repeating sulphonic acid functional groups, which are deprotonated and carry negative charge (ion). Thus, the ionized PSS can be used as a template to organize the other positively charged polymers (P3HT) via polaron formation and electrostatic interaction between the two materials as follows. (i) Initially, as the two molecules (P3HT and PSS) are close to each other in the organic solution, the hydrogen in the sulphonic acid groups of PSS is bound to a non-bonding electron pair of sulphur (S) atoms in P3HT, forming a R-SO 3 H···S hydrogen bond. 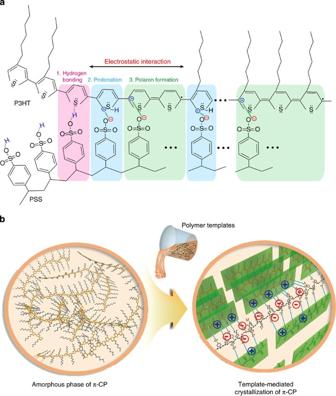Figure 6: Mechanism of the formation of TMC-induced fibril nanostructures. (a) Detailed mechanism of the electrostatic interaction between π-CPs (that is, P3HT) and the PSS template followed by hydrogen bonding, protonation and polaron formation in the solution state. (b) A schematic image of crystallized P3HT molecules along the PSS template via the electrostatic interaction between the P3HT and the template. (ii) The ionized proton (H + ) from PSS is transferred to a non-bonding electron pair of sulphur atoms in the polythiophene to form a sulphur cation, inducing an electrostatic interaction as follows: Figure 6: Mechanism of the formation of TMC-induced fibril nanostructures. ( a ) Detailed mechanism of the electrostatic interaction between π-CPs (that is, P3HT) and the PSS template followed by hydrogen bonding, protonation and polaron formation in the solution state. ( b ) A schematic image of crystallized P3HT molecules along the PSS template via the electrostatic interaction between the P3HT and the template. Full size image (iii) The protonated sulphur further changes the electronic structure within the thiophenes and thereby induces a radical cation (spin 1/2) on P3HT (P3HT + ) by emitting a hydrogen radical (H), which also induces an electrostatic interaction as follows: Critically, the structural repeat of the sulphonic-acid functionalized side-chain group along the single-bond carbon backbone can provide many electrostatic interactions for manipulating the P3HT orientation, which further act as crystal planes for nucleation on which the assembly of neighbouring P3HT molecules is energetically more favourable ( Fig. 6b ). Using a new TMC method, we succeed in inducing a structural orientation of π-CP along the template polymers over a long range to form an interconnected network throughout the π-CP films without being disconnected by the amorphous regions as in typical π-CPs. This achievement enables 3D isotropic transport with a similar order of improvement along the vertical and lateral directions. By monitoring the experiments with π-CPs and various doping/template agents, we identify that the bifunctional agent, PSS, incorporated in the light doping and template backbone would contribute to the formation of the well-connected nanomorphology of π-CP with TMC structures, leading to high-performance electronics exhibiting high on-currents and on/off ratios. Although many studies have been conducted on anisotropic alignment systems in π-CPs, our TMC-induced nanomorphology is fundamentally different from the simple chain-ordered structure that relies on the weak interchain interaction between π-CPs. In the TMC system, polymer templates can provide light doping and, as a result, a number of electrostatic interactions with π-CPs for manipulating the π-CP orientation, which enable superior charge transport along the crystallite nano-fibril structure in π-CP films. The achievement of a light doping and network formation of a crystallite nano-fibril structure of π-CPs via such a bifunctional polymer template indicates that a true interconnected pathway of π-CP with a 3D network formation can be prepared from the solution at RT. Because of the superior lateral and vertical charge transport of the TMC-induced π-CP films from the solution at RT, our approach represents an important step towards high-performance printable electronics using plastic substrates. Materials High-purity electronic-grade semiconducting P3HT polymers (~98%) were synthesized by Rieke Metals, MN, USA and were used as received. The regioregularity and average M w of the P3HT were ~92% and 53 kg mol −1 , respectively. The PDVT-10 polymer (average M w ≈50 kg mol −1 ) and DTS(PTTh 2 ) 2 small molecule were purchased from 1-material, Chemscitech Inc., QC, Canada. The insulating PSS template ( M w ≈75 kg mol −1 ) was purchased from Sigma-Aldrich and was dissolved in 18 wt% H 2 O with a pH of 1.55. Solution preparation To induce an electrostatic interaction between the semiconductors and the PSS template in solution, we directly added 10 mg of PSS (55.5 mg of the PSS solution) into a 10 mg ml −1 π-CP solution that was dissolved in a chloroform solvent. The final weight ratio of the organic semiconductor and the PSS template in the solutions was 1:1. For the DTS(PTTh 2 ) 2 small molecules, 2 mg of PSS (12 mg of the PSS solution) was introduced into a 10 mg ml −1 solution of the small molecules to attain a final weight ratio of 1:0.2. The solutions were subsequently stirred in the dark at RT for more than 72 h and were filtered through a 5-μm polytetrafluoroethylene filter. Film characterization Top-down TEM images of the sample films were recorded using a Tecnai G 2 F30 S-Twin microscope operated at an acceleration voltage of 300 kV. The sample films for TEM measurement were obtained by peeling the pre-deposited film ( t ≈70 nm) from a glass substrate, and the films were transferred onto 200-mesh copper grids (Electron Microscopy Sciences). GIWAXS measurements were performed at the 3C-SAXSl beam line in the Pohang Accelerator Laboratory (PAL) using a monochromatized X-ray radiation source of 10.55 eV ( λ =0.117 nm) and a two-dimensional charge-coupled device (CCD) detector (Mar165 CCD). The samples were mounted on a z -axis goniometer equipped with a vacuum chamber (~10 −3 torr), and the samples were 0.201 m away from the CCD detector. The incident angle of each X-ray beam was set as 0.6°, and the scattering angles were determined from the positions of the reflected X-ray beam from the silicon substrate using pre-calibrated silver beheaded. Device fabrication and characterization Before the deposition of the π-CP and π-CP:PSS solutions, heavily n-type-doped silicon substrates covered with 200-nm-thick SiO 2 were solicited with acetone and isopropyl alcohol, respectively, for 10 min and dried at 100 °C for 15 min. The π-CP and π-CP:PSS solutions were deposited onto the substrates at RT and ambient conditions, and the final thickness of the π-CP and π-CP:PSS layers was approximately 70 nm, as measured using a Surf Cored ET 3000. Top-contact and bottom-gate field-effect transistors were finalized with an Au source and drain electrode with a channel length of 50 μm and a width of 1,000 μm. To minimize the effect of environmental conditions, a thin polymethyl methacrylate film ( t ~40 nm) was deposited on the device before the measurement. For the large-area and flexible PFET, a 30-nm-thick aluminium layer was deposited as a gate electrode using a shadow mask on a polyethylene naphthalate substrate (4.4 × 4.4 cm 2 ). After spin casting a 5 wt% polyvinyl alcohol (PVA) aqueous solution mixed with ammonium dichromate onto the prepared substrate, we exposed and cross-linked the PVA gate insulator ( ε ≈5.4) using ultraviolet light for 90 s; the final film was rinsed with deionized water. The transfer and output characteristics were determined in a N 2 -filled glove box using a Keithley 4200 source metre (internal impedance>10 10 Ω). The saturation-regime mobility of the transistor was determined using the following equation: I ds =( W C i /2 L ) μ sat ( V g − V th ) 2 , where I ds is the source-drain current, C i (17.2 nF cm −2 ) is the capacitance per unit area, L is the channel length, W is the channel width, μ sat is the saturation-regime charge carrier mobility and V g and V th are the gate and threshold voltages, respectively. How to cite this article: Kwon, S. et al . Template-mediated nano-crystallite networks in semiconducting polymers. Nat. Commun. 5:4183 doi: 10.1038/ncomms5183 (2014).